Mutation in the seed storage protein kafirin creates a high-value food trait in sorghum Sustainable food production for the earth’s fast-growing population is a major challenge for breeding new high-yielding crops, but enhancing the nutritional quality of staple crops can potentially offset limitations associated with yield increases. Sorghum has immense value as a staple food item for humans in Africa, but it is poorly digested. Although a mutant exhibiting high-protein digestibility and lysine content has market potential, the molecular nature of the mutation is previously unknown. Here, building on knowledge from maize mutants, we take a direct approach and find that the high-digestible sorghum phenotype is tightly linked to a single-point mutation, rendering the signal peptide of a seed storage protein kafirin resistant to processing, indirectly reducing lysine-poor kafirins and thereby increasing lysine-rich proteins in the seeds. These findings indicate that a molecular marker can be used to accelerate introduction of this high nutrition and digestibility trait into different sorghum varieties. Sorghum ( Sorghum bicolor (L.) Moench) is a drought-tolerant C4 crop, one-third of which (~20 million tonnes of grain) is produced in the African continent from where it originates. Much of Africa has semi-arid, tropical or sub-tropical climate conditions in which maize cannot be grown because of water scarcity. Thus, its close relative, sorghum, has become the only viable food grain for many of the world’s most food-insecure people. Sorghum is also used as feed for animals in both developed and developing countries. One advantage of growing sorghum is that it usually does not compete for the lands, where other crops such as maize, wheat and rice can be grown. However, like other cereals, sorghum has poor protein quality because of lack of essential amino acids such as lysine and tryptophan [1] , [2] , [3] , [4] . Compounding this problem, sorghum proteins have very poor digestibility. These properties result in severe malnutrition when sorghum is consumed as the primary protein source [3] . The predominant seed proteins in sorghum are alcohol-soluble prolamins called kafirins. Kafirins comprise >70% of the total seed protein and serve as a repository of reduced nitrogen for breakdown and recycling into the proteins of the germinating seedling. Based on their molecular weight and sequence, they are classified into four classes, namely, α, β, γ and δ [5] , [6] . Similar to the maize zeins, kafirins are stored in the endoplasmic reticulum (ER) in spherical protein bodies (PBs), in which β- and γ-kafirins are located in the peripheral PB region and α- and δ-kafirins are encapsulated in the inner region [7] , [8] . The α-kafirins are the last proteins to be digested in the intestine and, because of their high abundance, the indigestibility reduces their nutritive value. The β- and γ-kafirins are rich in cysteine, which form disulphide bonds and are therefore assumed to block the accessibility of α-kafirins to hydrolytic enzymes [9] , [10] , [11] , [12] . A dominant floury mutant P721Q induced by chemical mutagenesis that exhibits significantly higher protein digestibility [13] has been shown to have market potential [14] . Furthermore, this mutant has a higher lysine content than the normal sorghum isoline, P721N [15] . The enhanced lysine level results mainly from an increase in lysine-rich non-kafirins, which further results from a slight decrease in lysine-deficient kafirins [14] . Like the o2 mutant in maize, this mutant has soft seed texture and is more susceptible to grain moulds. The o2 variant has been commercialized by selecting quantitative trait loci (QTLs) to overcome its inferior traits, resulting in the quality protein maize [16] , [17] . Correspondingly, a modified version of hdhl with harder endosperm has also been developed [18] . In the developing mutant endosperm, the PBs had irregular, invaginated shapes. It was hypothesized that the invagination of PBs resulted in expansion of their surface area to proteolytic enzymes, thereby increasing protein digestibility [12] . We sought to characterize the molecular basis of lysine and digestibility improvements to provide molecular markers for accelerated introgression into sorghum cultivars. Analogous to the sorghum phenotype, similar irregular and clumped PB morphologies in endosperm cells have previously been observed in two maize mutants with semi-dominant and dominant floury kernels [19] , [20] , [21] . These mutants resulted from point mutations at different sites in the ER signal peptides of a 22-kDa α-zein ( floury2 ) and a 19-kDa α-zein ( De-*B30 ). These mutations resulted in incorrectly processed mature zeins that remained tethered to the ER membrane [21] , [22] , [23] . Because of the phenotypic similarity, we hypothesized that the P721Q mutation in sorghum could be an aberrant kafirin. We used a pair of polymorphic SSR markers to follow the known locus of 22-kDa α-kafirin genes that we have cloned and characterized previously [24] . Indeed, we found that the polymorphic allele from P721Q was tightly linked to the floury phenotype in the F1 and BC1 populations. Because kafirin genes are the result of recent tandem amplification in the genome and are thus highly similar, we used random genomic and complementary DNA (cDNA) sequencing of 22-kDa α-kafirin genes and mRNAs in P721Q. Indeed, we identified a single mutant-specific kafirin gene copy that had a missense mutation in the signal peptide. To confirm that such a mutation renders the protein resistant to processing, we compared normal and mutant kafirin expression in transgenic maize. The mutant kafirin not only remained unprocessed in maize, but also triggered the unfolded protein response (UPR) and the formation of irregular PBs as observed in sorghum P721Q endosperm. Therefore, these results validate our direct approach to explain the mechanism of a valuable trait in agriculture and offer a molecular marker for introgressing such a trait into local germplasm, thereby increasing the acreage of more nutritious food. Genetic analysis of the mutant phenotype hdhl The highly digestible high-lysine ( hdhl ) mutant P721Q (Q for opaque) was generated by chemical mutagenesis (diethyl sulphate treatment) from P721N (N for normal) and exhibited kernels with a floury, non-vitreous phenotype [15] ( Fig. 1a ). The reduced accumulation of the main storage protein kafirins ( Fig. 1b ) in P721Q raised its lysine to a higher level than that of P721N [25] . To map hdhl , P721Q was crossed with Tx430 in reciprocal directions and all F1 seeds were floury, indicating that the action of hdhl is completely dominant. F1 seeds were subsequently self-pollinated or backcrossed to Tx430 as female, which gave rise to 3:1 segregation of floury and vitreous seeds in F2 and 1:1 in BC1, indicating that hdhl is a single locus. If the phenotype is caused by a mutation in the signal peptide of a kafirin gene, we could determine whether it is linked to these genes and whether one of its copies has such a specific mutation. We previously determined by comparative genomics that all 20 α-kafirin genes were clustered on Chr. 5 of the BTx623 genome [26] . SSR markers were designed based on the BAC SB40L16 sequence, which comprises a cluster of 10 active 22-kDa α-kafirin genes of Btx623 within 35 kb, a sorghum chromosome segment that, as a whole, became integrated in the maize genome by transformation [27] . Transgenic maize seeds expressed and processed kafirins properly and served as a positive control in our experiments below. 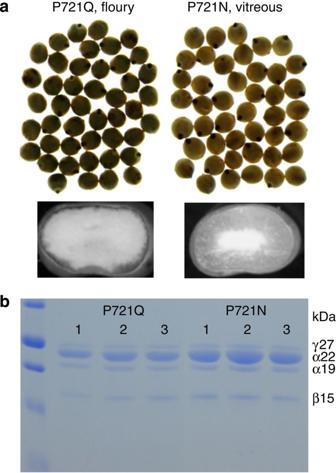Figure 1: Characterization of the phenotype of the highly digestible high-lysine mutant. (a) Seed phenotype of P721Q and P721N. (b) Kafirin accumulation patterns of P721Q and P721N analysed by SDS–PAGE. Protein markers in the leftmost lane from top to bottom are 37, 25, 20, 15 and 10 kDa. Total kafirin loaded in each lane was equal to 200 μg of sorghum flour. The size for each band is indicated. Figure 1: Characterization of the phenotype of the highly digestible high-lysine mutant. ( a ) Seed phenotype of P721Q and P721N. ( b ) Kafirin accumulation patterns of P721Q and P721N analysed by SDS–PAGE. Protein markers in the leftmost lane from top to bottom are 37, 25, 20, 15 and 10 kDa. Total kafirin loaded in each lane was equal to 200 μg of sorghum flour. The size for each band is indicated. Full size image Although there were other 22-kDa α-kafirin genes within a million base pairs on the same chromosome [26] , the selected SSR markers showed that the tandem kafirin cluster on BAC SB40L16 was tightly linked to seed floury and vitreous phenotypes and the recombination frequency was <1% ( Fig. 2 and Table 1 ). We used universal primers based on the conserved 5′-UTR and 3′-end of the coding sequence (CDS) regions of the 22-kDa α-kafirin gene cluster to amplify, from genomic DNA, all copies from P721N and P721Q for sequencing with ABI-3730 capillary electrophoresis. We found that seven out of 77 sequences had a single nucleotide G→A substitution at position 61 relative to the first nucleotide of the start codon ( Fig. 3 ), whereas no such mutation was found in 96 sequences from P721N. Because we previously had already indicated that all 10 kafirin genes in the cluster are expressed [27] , these results would be consistent with one out of 10 gene copies of the kafirin cluster producing the mutant protein. We also analysed cDNA sequences of the 22-kDa α-kafirin genes from their developing endosperms and confirmed that the mutant transcript was only present in P721Q (five out of 96). This missense mutation results in the last amino acid alanine (Ala) in the signal peptide being replaced with threonine (Thr) ( Fig. 4 ). 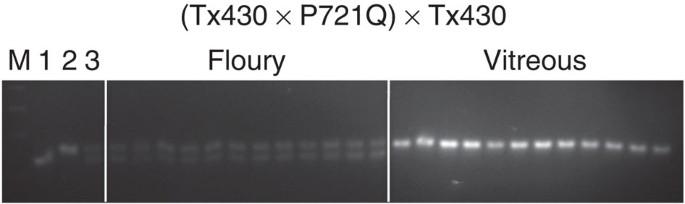Figure 2: Linkage analysis of the floury phenotype with a SSR marker from Chr. 5 near to the 22-kDa α-kafirin cluster. The floury progeny seeds all contained the lower band originated from p721Q, whereas the vitreous progeny uniformly yielded the single band from Tx430. M: DNA markers from top to bottom are 400, 300, 200 and 100 bp; lane 1, P721Q; lane 2, Tx430; lane 3, F1 of Tx430 × P721Q. Figure 2: Linkage analysis of the floury phenotype with a SSR marker from Chr. 5 near to the 22-kDa α-kafirin cluster. The floury progeny seeds all contained the lower band originated from p721Q, whereas the vitreous progeny uniformly yielded the single band from Tx430. M: DNA markers from top to bottom are 400, 300, 200 and 100 bp; lane 1, P721Q; lane 2, Tx430; lane 3, F1 of Tx430 × P721Q. Full size image Table 1 Linkage analysis of the selected marker near the α-kafirin locus on Chr. 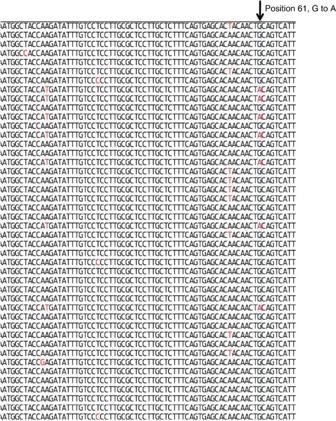Figure 3: Partial alignment of the 22-kDa α-kafirin cluster amplified from P721Q genomic DNA. The position of the G→A substitution is marked with the downward arrow. 5 and the seed phenotype Full size table Figure 3: Partial alignment of the 22-kDa α-kafirin cluster amplified from P721Q genomic DNA. The position of the G→A substitution is marked with the downward arrow. 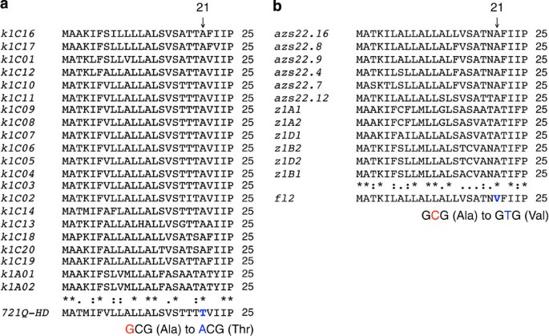Figure 4: Missense mutation at the 21st amino acid of the signal peptide in P721Q-hdhland maizefloury2mutants. The missense mutation is marked with an arrow at the 21st amino acid of the signal peptide in P721Q-hdhl(a) and maizefloury2(b). (a) P721Q-hdhlharbouring the G→A transition resulted in Ala being replaced with Thr; (b) maizefloury2containing C→T transition caused the replacement of Ala with Val. Full size image Figure 4: Missense mutation at the 21st amino acid of the signal peptide in P721Q- hdhl and maize floury2 mutants. The missense mutation is marked with an arrow at the 21st amino acid of the signal peptide in P721Q- hdhl ( a ) and maize floury2 ( b ). ( a ) P721Q- hdhl harbouring the G→A transition resulted in Ala being replaced with Thr; ( b ) maize floury2 containing C→T transition caused the replacement of Ala with Val. Full size image Conservation of α-prolamin signal peptides in Panicoideae The α-kafirins and α-zeins arose late in the evolution of the prolamins and have been found in the subfamily of the Panicoideae that include the sequenced genomes of foxtail millet, sorghum and maize [24] . Their signal peptide is 21 amino acids long and is cleaved when the protein is transported into the inner side of PB for storage. The Ala at position 21 is critical for cleavage, as it is conserved in all 19- and 22-kDa α-prolamins in foxtail millet, sorghum, coix and maize ( Fig. 5 ). In the floury2 mutant of maize, the same Ala is replaced with valine (Val) in a 22-kDa alpha zein ( Fig. 4 ), resulting in the retention of the signal peptide at maturity. As a consequence, the immature zein is tethered to the PB membrane, resulting in irregular PBs. When signal peptides from α-prolamins of species of the Panicoideae such as maize, coix, sorghum, sugarcane and pearl millet were aligned, only three amino acids were completely conserved except for the start codon, leucine at positions 11 and 14 and Ala at 21 ( Fig. 5 ). 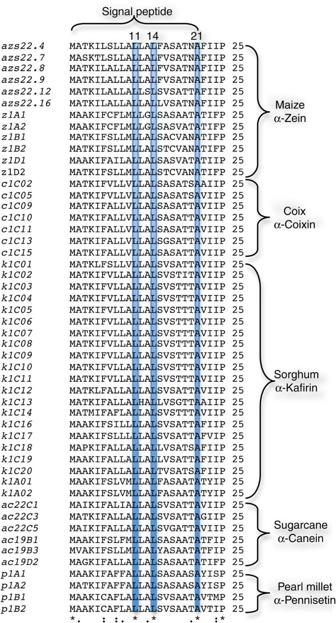Figure 5: Alignment of the signal peptides of α-prolamins from the grass subfamily. Three amino acids at positions 11, 14 and 21 are highly conserved except for the start codon. Figure 5: Alignment of the signal peptides of α-prolamins from the grass subfamily. Three amino acids at positions 11, 14 and 21 are highly conserved except for the start codon. Full size image Phenocopying of irregular PBs in maize with kafirin mutant To demonstrate that this mutation indeed renders the kafirin resistant to signal peptide processing, we took advantage of the transgenic maize line as a control, in which we expressed the normal kafirin cluster [27] . We wanted to use a heterologous system to exclude any other sorghum protein and sequence in this test. Using only the mutant sorghum transcript under the control of the maize 22-kDa α-zein promoter, we transformed maize with the mutant gene construct. The construct was also coupled with the visible GFP marker driven by the 10-kDa δ-zein promoter to facilitate scoring of positive progeny seeds ( Fig. 6a ). At 18 days after pollination (DAP), a number of immature kernels were collected and these segregated 1:1 for green and non-green seeds. The null segregant and positive transgenic endosperms were used to extract RNA. Reverse transcription (RT)-PCR analysis confirmed that the green seeds highly expressed the mutant sorghum allele ( Fig. 6b ). Furthermore, western blot analysis with a 22-kDa α-zein antibody showed that in transgenic maize harbouring the mutant kafirin gene, a slower migrating protein band (24 kDa) above the processed 22-kDa α-zein is visible. This band is absent in the control with the normal kafirin genes in separate transgenic maize lines ( Fig. 6c ). Moreover, a transacting gain of function was observed. Expression of the Bip gene was significantly enhanced, indicating that the unprocessed kafirin induces the UPR in maize ( Fig. 6d ). As a consequence, the levels of the 22-kDa α-zeins were noticeably reduced compared with the null segregants ( Fig. 6c ), consistent with the observation in P721Q ( Fig. 1b ) and the UPR-induced translational repression. 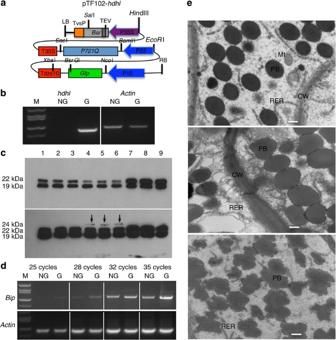Figure 6: Expression of mutant and normalkafiringenes in maize. (a) pTF102-mutant kafirin construct. (b) RT-PCR analysis of the expression of mutant kafirin in maize endosperm at 18 DAP. NG, non-green (null segregant); G, green (mutant kafirin); M, DNA markers from top to bottom are 2, 1.5, 1.4, 1 and 0.75 kb. (c) Western blot analysis of kafirin accumulation. Highly diluted protein loaded in each lane represents prolamins extracted from 0.5 μg maize flour. The antiserum can crossreact with the 22-kDa α-zeins/kafirins and 19-kDa α-zeins. The unprocessed mutant 22-kDa α-kafirin (24 kDa) migrated slower than the 22-kDa α-zeins and normal 22-kDa α-kafirins, as indicated by arrows. Upper panel, the film exposed for 10 s; bottom panel, the film exposed for 75 s. Lanes 1–3, null segregants without GFP expression; lanes 4–6, mutant kafirin transgenic seeds with GFP expression; lanes 7–9, transgenic seeds expressing normal 22-kDa α-kafirins. (d) RT-PCR analysis of the expression of theBipgene. M, DNA markers from top to bottom are 2, 1.5, 1.4, 1 and 0.75 kb. Theactingene served as a control. (e) Transmission electron micrographs of PBs in null segregant (upper panel), maize transformed with normal kafirins (middle panel) and mutant kafirin (bottom panel) endosperms at 18 DAP. CW, cell wall; RER, rough endoplasmic reticulum; Mt, mitochondria. Scale bar, 500 nm. Figure 6: Expression of mutant and normal kafirin genes in maize. ( a ) pTF102-mutant kafirin construct. ( b ) RT-PCR analysis of the expression of mutant kafirin in maize endosperm at 18 DAP. NG, non-green (null segregant); G, green (mutant kafirin); M, DNA markers from top to bottom are 2, 1.5, 1.4, 1 and 0.75 kb. ( c ) Western blot analysis of kafirin accumulation. Highly diluted protein loaded in each lane represents prolamins extracted from 0.5 μg maize flour. The antiserum can crossreact with the 22-kDa α-zeins/kafirins and 19-kDa α-zeins. The unprocessed mutant 22-kDa α-kafirin (24 kDa) migrated slower than the 22-kDa α-zeins and normal 22-kDa α-kafirins, as indicated by arrows. Upper panel, the film exposed for 10 s; bottom panel, the film exposed for 75 s. Lanes 1–3, null segregants without GFP expression; lanes 4–6, mutant kafirin transgenic seeds with GFP expression; lanes 7–9, transgenic seeds expressing normal 22-kDa α-kafirins. ( d ) RT-PCR analysis of the expression of the Bip gene. M, DNA markers from top to bottom are 2, 1.5, 1.4, 1 and 0.75 kb. The actin gene served as a control. ( e ) Transmission electron micrographs of PBs in null segregant (upper panel), maize transformed with normal kafirins (middle panel) and mutant kafirin (bottom panel) endosperms at 18 DAP. CW, cell wall; RER, rough endoplasmic reticulum; Mt, mitochondria. Scale bar, 500 nm. Full size image The level of the mutant kafirin in comparison with the total α-zein is relatively low, but it was previously shown that the dominant-negative 19-kDa α-zein in the De-*B30 mutant induces dramatic PB alterations and UPR with very low levels of accumulation [21] . Nevertheless, we wondered whether the mutant protein is sufficient to trigger a deformation of PBs as it has been observed in P721Q. Therefore, transmission electron microscopy (TEM) examination was also performed with endosperms of maize from transgenic and non-transgenic lines. Indeed, this low level of the mutant kafirin gave rise to PBs that were all irregular and frequently clumped, whereas the PBs of maize transformed with non-mutant kafirins and the null-segregant control showed normal phenotype ( Figs 6e and 7 ). Therefore, we showed that the coding region of the mutant gene, which is tightly linked to the PB phenotype in sorghum P721Q, produces the same phenotype in maize as a gain of function. This also confirmed that as in floury2 in maize [20] , the compartmentalization of storage proteins in PBs is conserved between the two species. 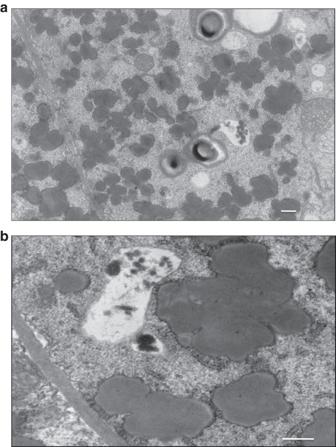Figure 7: Transmission electron micrographs of PBs in maize endosperm transformed with mutant kafirin at 18 DAP. (a) View at low magnification. (b) View at higher magnification. Scale bar, 500 nm. Figure 7: Transmission electron micrographs of PBs in maize endosperm transformed with mutant kafirin at 18 DAP. ( a ) View at low magnification. ( b ) View at higher magnification. Scale bar, 500 nm. Full size image We have taken a direct approach to investigate a valuable trait in agriculture. A cereal such as sorghum can substitute for maize in areas with low water supply and serve those geographical areas with food. Sorghum also has high nitrogen utilization efficiency, thereby cutting expenses in fertilizer [28] . However, if seed proteins lack digestibility and certain essential amino acids, it would have to be supplemented by other crops that lack drought resistance and require energy-costly nitrogen, such as soya beans. Instead of supplementation, a stand-alone diet with sorghum would be desirable. Therefore, a lysine-enhanced and highly digestible sorghum variety has gained broad attention. Nevertheless, similar to quality protein maize, hdhl requires additional selection to identify modifier genes that make the mutant kernels harder [29] . As shown in maize, the introduction of such different mutations into local germplasm is a complex and time-consuming process [30] . Unlike P721Q and floury2 , the seed phenotype of the transgenic maize expressing the mutant kafirin is vitreous. This difference between hdhl sorghum and transgenic maize shows that disruption of PB structure and induction of UPR per se do not necessarily induce endosperm opacity. On the contrary, residual levels of zeins are apparently high enough to produce normal endosperm texture. The same observation was made when RNA interference was used to reduce α-zeins in two types of maize. It was shown that non-vitreous phenotypes could be overcome with a certain threshold of residual α-prolamin synthesis. In normal maize, reduction of α-zeins gave rise to non-vitreous, high-lysine kernels, but in Illinois High Protein reduction of α-zeins with RNA interference left enough α-zeins to give rise to vitreous high-lysine kernels [31] . Given the variability of the phenotype and with the introduction of modifiers for kernel hardness, breeders cannot rely on phenotype for the introgression of combined traits into local germplasms. Using a single molecular marker to follow the point mutation in the signal peptide of the mutant kafirin will allow breeders to select their material without relying on a phenotype. Plant materials Gebisa Ejeta and Bruce Hamaker at Purdue University generously provided sorghum normal and hdhl seeds P721N and P721Q. P721Q was crossed to Tx430, resulting in an F1; then F1 progeny were self-pollinated and backcrossed to Tx430 as female. Maize Hi-II B and A lines for transformation and the transgenic lines expressing normal kafirins were our own materials. Genetic analysis The SSR marker (SSR-F: 5′-AGTCAACAACTCCCTCCACC-3′; SSR-R: 5′-ATCGGCTGGTCGTCGACTGAG-3′) for segregation analysis was designed near the first 22-kDa α-kafirin gene in the BAC SB40L16. In total, 44 samples for each floury and vitreous seed from BC1 and 25 for each from F2 were extracted for genotyping genomic DNA. Genomic and cDNA sequencing of the 22-kDa α-kafirin genes A universal primer pair priming in the 5′-UTR and at the 3′-end of coding region of the 22-kDa α-kafirin genes (k1CF: 5′-CAACGTCCTCACAACAATGGC-3′; k1CR: 5′-TCCAACGATGGGTTGCTGCCA-3′) was used to amplify all non-truncated kafirins from genomic DNA and endosperm cDNA from P721N and P721Q. PCR products from genomic DNA were cloned into T-easy vector (Promega) and 96 colonies for each sample were picked to sequence on ABI-3730. For cDNA sequencing, RNA was extracted from whole-developing sorghum grains from self-pollinated (18–22 DAP) P721N and P721Q plants, and DNase-treated and cDNA-synthesized according to a previously described method [32] . The α-kafirin cDNAs were amplified using the above primers and cloned into pJET (Fermentas). A total of 96 α-kafarin clones, confirmed with colony PCR, were sequenced from P721N and P721Q with universal pJET primers and aligned using Codon-code Alligner. Maize transformation The mutant 22-kDa α-kafirin copy was driven by the maize 22-kDa α-zein promoter and coupled to the visible GFP marker driven by the maize 18-kDa δ-zein promoter. The two gene cassettes were inserted into the binary vector pTF102 ( Fig. 6a ). About 200 immature embryos (1.5–2.0 mm), collected around 10 DAP from crosses of Hi-II B and A lines, were dissected for transformation [33] . After two rounds of selection with bialaphos, the fast-growing and friable calli were subjected to regeneration. The positive transformation events could be confirmed by PCR with the primer pair k1CF and k1CR as described above. RT-PCR Total RNA was extracted by using TRIzol reagent (Invitrogen). A total of 5 μg RNA was digested with DNase I (Invitrogen) and then reverse transcribed. hdhl primer pair has been mentioned above; the Actin and Bip gene primer pairs were Actin-F, 5′-GCCGGTTTCGCTGGTGATGATGCGCC-3′; Actin-R, 5′-GTGATCTCCTTGCTCATACGATCGGC-3′, and Bip-F, 5′-TTGTTCGCGTTTTCAGTTGC-3′; Bip-R, 5′-CACGACGAGCTGTAGATGGTT-3′. Western analysis Prolamins were extracted according to a previously described method [34] and separated on 15% polyacrylamide SDS–PAGE gels, transferred to nitrocellulose and probed with total rabbit α-zein antiserum at 1/10,000 dilution. Secondary antibody was horse radish peroxidase-conjugated goat anti-rabbit (Pierce) used at 1/5,000 dilution, and the detection was done with the West Pico chemiluminescent detection system (Pierce). Transmission electron microscopy Two-millimetre thick sections were sliced perpendicular to the aleurone layer in order to include the pericarp, aleurone and 10–20 cell layers of the endosperm. All these slices were fixed in 5% glutaraldehyde in 0.1 M sodium cacodylate buffer, pH 7.4, containing 2% sucrose in a 2 ml tube. Samples were fixed overnight at 4 °C and for another 3 h at room temperature. The tissues were rinsed for 2–3 h with several changes of 0.1 M sodium cacodylate buffer containing decreasing amounts of sucrose. They were then post-fixed in buffered 1% Osmium Tetroxide at 4 °C overnight followed by dehydration in a graded series of acetone and embedded in Epon resin. Ninety-millimetre thin sections were cut on a Leica EM UC6 ultramicrotome using a diamond knife. Sectioned grids were stained with a saturated solution of uranyl acetate and lead citrate. Sections were viewed at 80 Kv with a Philips CM 12 transmission electron microscope. Accession code: The sequence of mutant kafirin has been deposited in Genbank under accession code KF141792 . How to cite this article: Wu, Y. et al. Mutation in the seed storage protein kafirin creates a high-value food trait in sorghum. Nat. Commun. 4:2217 doi: 10.1038/ncomms3217 (2013).